High-capacity antimony sulphide nanoparticle-decorated graphene composite as anode for sodium-ion batteries Sodium-ion batteries are an alternative to lithium-ion batteries for large-scale applications. However, low capacity and poor rate capability of existing anodes are the main bottlenecks to future developments. Here we report a uniform coating of antimony sulphide (stibnite) on graphene, fabricated by a solution-based synthesis technique, as the anode material for sodium-ion batteries. It gives a high capacity of 730 mAh g −1 at 50 mA g −1 , an excellent rate capability up to 6C and a good cycle performance. The promising performance is attributed to fast sodium ion diffusion from the small nanoparticles, and good electrical transport from the intimate contact between the active material and graphene, which also provides a template for anchoring the nanoparticles. We also demonstrate a battery with the stibnite–graphene composite that is free from sodium metal, having energy density up to 80 Wh kg −1 . The energy density could exceed that of some lithium-ion batteries with further optimization. Lithium-ion batteries (LIBs) have been the main energy storage medium for mobile applications for the past 20 years. There has been growing focus on energy storage for larger application such as electric vehicle and stationary storage for renewable energies. Sodium-ion batteries (NIBs) are an alternative to LIBs for these applications because of the lower cost and larger abundance of Na, and therefore have recently attracted much attention [1] , [2] . One of the main obstacles to the commercialization of NIBs is the limited choice of anode materials that can provide good stability and high-rate performance [3] . Commercialization of the LIBs was mainly driven by the ability for lithium to intercalate into graphite, resulting in large and stable capacity. As opposed to lithium, sodium cannot be intercalated into graphite [4] , [5] . Hard carbon and carbon fibres were discovered as possible anodes for NIBs [6] , [7] , [8] , [9] , [10] ; however, stable capacity is only up to about 250 mAh g −1 . Recently, there has been development on using metallic and intermetallic materials as anodes for NIBs [11] , [12] , [13] , [14] , [15] , [16] , [17] , [18] . For example, Na can alloy with Sn and Sb to form Na 15 Sn 4 and Na 3 Sb, respectively, resulting in a theoretical capacity of 847 mAh g −1 and 660 mAh g −1 . Komaba et al. [17] have demonstrated that Na can be alloyed with Sn with a charge capacity of about 800 mAh g −1 , close to the theoretical capacity of Sn. However, in order to keep the stability of the material, Sn has to be cycled between 0 and 0.8 V, resulting in a reversible capacity of only 500 mAh g −1 at a rate of 50 mA g −1 . Qian et al. [12] have reported nanocomposite Sb/C that could have a capacity of about 600 mAh g −1 at a rate of 100 mA g −1 , where the capacity decreased to 382 mAh g −1 at a rate of 1,500 mA g −1 . On the other hand, oxide materials such as SnO 2 [19] , [20] , and Sb 2 O 4 [21] , were also reported as anode materials for NIBs. Su et al. [20] have obtained SnO 2 @graphene with a charge capacity of above 700 mAh g −1 at a rate of 20 mA g −1 . Sun et al. [21] have shown reversible capacity of 896 mAh g −1 for Sb 2 O 4 at a rate of 1/70C, but capacity was much reduced at a higher current rate (the capacity decreases to 143 mAh g −1 at a rate of 640 mA g −1 ). Moreover, an intrinsic problem of oxide materials is the irreversibility of the Na 2 O formation with a low first cycle efficiency of typically around 30–40%, resulting in a fraction of the Na in the anode material that is not reusable. Thus, there is a need for the development of materials with improved first cycle efficiency that can give higher capacity at higher current. Previous work by Wu et al. [22] demonstrated a reversible capacity of 664 mAh g −1 at 20 mA g −1 and 350 mAh g −1 at 800 mA g −1 for Sn–SnS–C nanocomposites. Herein, we have investigated the use of Sb 2 S 3 as anode material for NIBs. In LIBs, Sb 2 S 3 first undergoes a conversion reaction between the sulphide and lithium, followed by a metal alloying reaction with lithium [23] . On the basis of similar mechanisms, the reactions between Sb 2 S 3 and sodium are expected as below: One can get 12 moles of electron and Na + ion storage per mole of Sb 2 S 3 , resulting in a theoretical capacity of 946 mAh g −1 . The potential advantages of Sb 2 S 3 over Sb for Na insertion are: higher theoretical capacity than Sb (660 mAh g −1 ) because of the lower weight of the S atoms, as well as an expected improvement in mechanical stability due to smaller volume change during charge and discharge from the sulphides. Moreover, sulphides formation is typically more reversible than oxides, resulting in a higher first cycle efficiency than oxide materials. Bulk Sb 2 S 3 can accommodate about 12 Na atoms during the first discharge, but less than half of the Na can be extracted. It is therefore essential to reduce the particle size to reduce Na ionic pathway and form a composite with graphene layers to enhance the electrical connectivity of the material in order to fully utilize the potential of the Sb 2 S 3 material. In the present study, we develop a chemical synthesis routine via deposition of peroxoantimonate from hydrogen peroxide-rich solution and its subsequent sulphurisation with hydrogen sulphide to form a conformal coating of nanocrystallite stibnite (Sb 2 S 3 ) onto reduced graphene oxide (rGO). The composite material performs extremely well as the anode for NIB. About 9.2 Na (730 mAh g −1 ) can be reversibly inserted and removed from the material at a rate of 50 mA g −1 (about 0.067C). The material retains its charge capacity even at higher current rates. When the current rate is increased to 1,500 mA g −1 (about 2.5C), charge capacity of 610 mAh g −1 can be obtained. Even when the current is increased to 3,000 mA g −1 , >70% of the capacity (520 mAh g −1 ) can still be used, which corresponds to a charge and discharge time of 10 min. This would allow fast charging of NIBs in the future. In addition to the excellent rate capability, the material also shows stable cycle performance. Capacity retention is >95% after 50 cycles at 50 mA g −1 . The enhanced rate capability and cycle stability of the materials are attributed to the intimate contact of stibnite to the reduced graphene sheets that provides a structure for electrical conductivity as well as a platform for anchoring the nanoparticles. The anode material is also coupled with a Na 2/3 Ni 1/3 Mn 2/3 O 2 cathode to form a Na metal-free full cell. The full cell demonstrates an energy density of 80 Wh kg −1 and shows good cycle performance. Material synthesis and characterization The rGO/Sb 2 S 3 composite featured in this study was fabricated by sulphurisation of peroxoantimonate-coated graphene oxide (GO) in alcohol and subsequent vacuum annealing at 300 °C (ref. 24 ). Formation of crystalline Sb 2 S 3 was confirmed by X-ray diffraction (XRD) analysis. The amount of carbon content in the composite is determined to be about 17 wt% by elemental analysis. 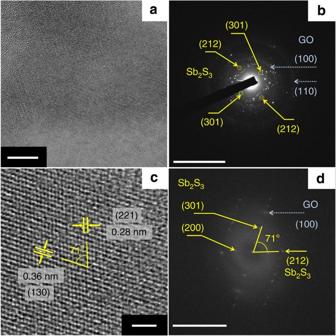Figure 1: TEM images and SAED pattern of antimony sulphide-coated GO. (a) TEM image (scale bar, 10 nm) and (b) the corresponding SAED pattern (scale bar, 10 nm−1). (c) Magnified section of the TEM image with the corresponding crystal lattice fringes (scale bar, 2 nm). (d) FFT of the TEM image is depicted in frame (scale bar, 5 nm−1). Figure 1a–d shows the transmission electron microscopy (TEM) micrograph of the as-synthesized Sb 2 S 3 -coated GO (a). The selected area electron diffraction (SAED) shows the diffraction pattern of polycrystalline Sb 2 S 3 with the characteristic pattern of stibnite. Fast Fourier transform (FFT) of the high-resolution TEM of Sb 2 S 3 is shown in frame (d), with the few diffraction planes of stibnite. The diffraction patterns of the GO are clearly shown in the FFT as well as in the SAED pattern. The crystalline size as deduced from TEM studies is between 15 and 30 nm and the average crystallite size of antimony sulphide calculated by Scherrer equation based on the X-ray powder diffraction is 16 nm. Figure 1: TEM images and SAED pattern of antimony sulphide-coated GO. ( a ) TEM image (scale bar, 10 nm) and ( b ) the corresponding SAED pattern (scale bar, 10 nm −1 ). ( c ) Magnified section of the TEM image with the corresponding crystal lattice fringes (scale bar, 2 nm). ( d ) FFT of the TEM image is depicted in frame (scale bar, 5 nm −1 ). Full size image Electrochemical properties Electrodes were made by mixing active materials with acetylene black and carboxymethyl cellulose (CMC) sodium salt in de-ionized water in the ratio 6:2:2. The electrode was made into 2016 coin cells with sodium metal as the counter electrode. One molar NaClO 4 in propylene carbonate with 5 wt% fluorinated ethylene carbonate (FEC) was used as the electrolyte. FEC was added to improve the stability of the material with cycling [12] , [25] (see Supplementary Fig. S1 for comparison between electrolyte with and without FEC). Reference electrodes with Cu:AB:CMC=6:2:2 and graphene:AB:CMC=6:2:2 were also tested under the same condition, showing small contributions to the capacity due to carbon black, binder and graphene. In addition, bulk Sb 2 S 3 from Sigma-Aldrich with a particle size of about 10 μm was also tested for comparison. rGO/Sb 2 S 3 electrodes show a first discharge capacity of 1,050 mAh g −1 (see Fig. 2a ). Only a small contribution of the discharge capacity is due to graphene (162 mAh g −1 ), carbon black and binder (43 mAh g −1 ) (see Supplementary Discussion and Supplementary Fig. S2 for detailed calculations). Thus, the capacity that originates from insertion of Na into Sb 2 S 3 is 845 mAh g −1 , which is close to full utilization of the Sb 2 S 3 active material. On the other hand, first charge capacity of rGO/Sb 2 S 3 is 730 mAh g −1 (9.2 Na), out of which only 38 mAh g −1 and 8 mAh g −1 come from graphene and carbon black, respectively. Overall, the first cycle efficiency of the rGO/Sb 2 S 3 electrodes is 69.2%, which is higher than that of metal oxides such as SnO 2 . During charge and discharge, 9.2 Na can be reversibly inserted and extracted from the electrode. In contrast, commercial bulk Sb 2 S 3 (Sigma-Aldrich) with a particle size of about 10 μm shows a first cycle discharge and charge capacity of 980 and 337 mAh g −1 , respectively, corresponding to a first cycle efficiency of 34.4% (see Fig. 2a ). rGO/Sb 2 S 3 shows a much higher reversible capacity than bulk Sb 2 S 3 even though the first discharge capacity is similar. 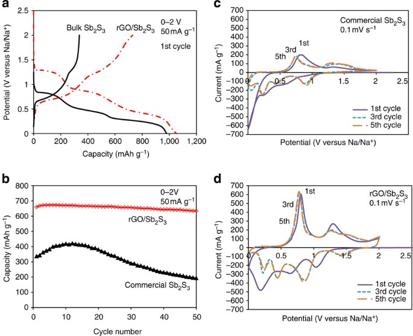Figure 2: Electrochemical performance of bulk Sb2S3and rGO/Sb2S3. (a) First cycle charge–discharge profiles at 50 mA g−1, (b) cycle performance at 50 mA g−1, (c) cyclic voltammogram of bulk Sb2S3and (d) cyclic voltammogram of rGO/Sb2S3. Figure 2: Electrochemical performance of bulk Sb 2 S 3 and rGO/Sb 2 S 3 . ( a ) First cycle charge–discharge profiles at 50 mA g −1 , ( b ) cycle performance at 50 mA g −1 , ( c ) cyclic voltammogram of bulk Sb 2 S 3 and ( d ) cyclic voltammogram of rGO/Sb 2 S 3 . Full size image To understand the main difference between rGO/Sb 2 S 3 and bulk Sb 2 S 3 electrodes, cyclic voltammetry at a scan rate of 0.1 mV s −1 were carried out on the two electrodes. Results are shown in Fig. 2c,d . The profiles during the first cycle for both electrodes are distinctively different from subsequent cycles, suggesting that there is an activation step during the first discharge. During second and subsequent cycles, both bulk Sb 2 S 3 and rGO/Sb 2 S 3 electrodes show reduction peaks around 0.25, 0.45 and 0.9 V versus Na/Na + and oxidation peaks around 0.73 and 1.3 V versus Na/Na + . The reduction and oxidation potentials at 0.25/0.45 and 0.73 V agree well with the potential positions of alloying of Sb with Na [12] . The potential pair at 0.9/1.3 V is attributed to conversion reaction with sulphur atoms in the material. rGO/Sb 2 S 3 shows enhanced reaction currents for both alloying and conversion reactions, which is the main reason the overall reversible capacity is higher. The role of graphene on the electrochemical performance was investigated by comparing the activity of nanocrystalline Sb 2 S 3 without graphene (n-Sb 2 S 3 ) synthesized by a co-precipitation method with rGO/Sb 2 S 3 and bulk Sb 2 S 3 (see Supplementary Fig. S3 ). n-Sb 2 S 3 shows a first cycle charge capacity of 503 mAh g −1 , larger than the charge capacity of bulk Sb 2 S 3 but smaller than that of rGO/Sb 2 S 3 . Reversible capacity is higher by reducing the particle size, but graphene templating is needed to further enhance the reversible capacity from the reaction by allowing more effective de-alloying and recombination of the metal-sulphide during sodium removal. Figure 2b shows the cycle performance of both bulk Sb 2 S 3 and rGO/Sb 2 S 3 at a current rate of 50 mA g −1 . Capacity of bulk Sb 2 S 3 increases from 337 to 419 mAh g −1 during the first 10 cycles, but decreases afterwards to <200 mAh g −1 after 50 cycles, <50% of the maximum capacity. The increase in capacity during the initial 10 cycles for bulk Sb 2 S 3 is accompanied by a cycle efficiency of above 100%, meaning that this is due to an increase in extraction of Na from the electrode that is originally inserted during the first discharge. However, cycle efficiency settles down to about 97.2% with prolonged cycling, and the capacity reduction is caused by the loss of active material. In contrast, rGO/Sb 2 S 3 shows a capacity of about 670 mAh g −1 , with a capacity retention of >95% after 50 cycles. Cycle efficiency is about 98.7% for rGO/Sb 2 S 3 , suggests less loss per cycle compared with bulk material. In addition to the excellent cycle stability, rGO/Sb 2 S 3 also shows good high-rate capability. The electrode was discharged and charged at a rate of 50, 100, 250, 500, 1,000, 1,500, 2,000 and 3,000 mA g −1 for five cycles each. After the rate test, the electrode was tested again at 50 mA g −1 to investigate the effect of rate test on the stability of the electrode. Detailed plot of the charge capacity versus cycle number is given in Supplementary Fig. S4 . The charge capacities at different current rates are summarized in Fig. 3b . In addition to the high capacity at low rate, a charge capacity of 611 mAh g −1 can be obtained at a current rate of 1,500 mA g −1 , which corresponds to a charge and discharge time of about 24 min (2.5C). When the current rate is increased to 3,000 mA g −1 , a capacity of 520 mAh g −1 can still be obtained (>70% of the available 730 mAh g −1 at a low current rate). This corresponds to a charge and discharge time of 10 min (6C), sufficient for high-rate applications such as electric vehicles and power tools. The high-rate capability indicates that the electrode materials allow fast transfer of Na and electrons through our material design. 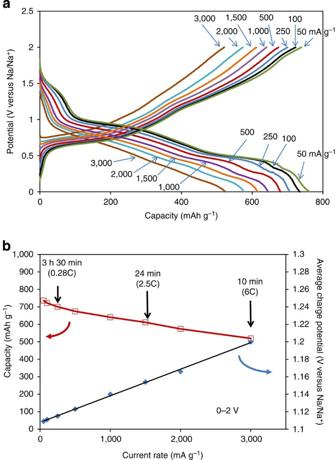Figure 3: Rate performance of rGO/Sb2S3. (a) Charge–discharge curves of rGO/Sb2S3at different current rates and (b) respective capacity and average charge potential at different current rates. Figure 3a shows selected charge–discharge curves at different current rates. There is minimal increase in polarization even at high current rate of 3,000 mA g −1 , suggesting good electrical connectivity with the graphene template. Average charge potentials of the electrode at different current rates are shown in Fig. 3b , indicating that the working potential only increases by 0.05 V when the current is increased from 50 to 1,500 mA g −1 , an increase of 30 times the current and by 0.1 V when the current is increased to 3,000 mA g −1 . The stability of the electrode was verified again after rate test. When the current rate is reduced back to 50 mA g −1 after the rate test, the initial capacity is restored (see Supplementary Fig. S4 ). Figure 3: Rate performance of rGO/Sb 2 S 3 . ( a ) Charge–discharge curves of rGO/Sb 2 S 3 at different current rates and ( b ) respective capacity and average charge potential at different current rates. Full size image The intimate contact between the antimony sulphide and the rGO is partly responsible for the enhanced behaviour of the NIB anode. The small polarization at high current rate is an indication of good electronic connectivity within the graphene composite. The small particle size (15–30 nm from TEM) allows fast Na movement into and out of the particles during charge and discharge. To further elucidate the charge–discharge process, XRD and scanning electron microscopy (SEM) of the electrodes were taken at different states of charge during the first cycle: (i) half discharged to 1 V, (ii) fully discharged to 0 V, (iii) fully discharged to 0 V and then charged to 2 V. The cells were then disassembled in a glove box, washed with dimethyl carbonate to remove the salt, and then sealed in wax for XRD measurement. 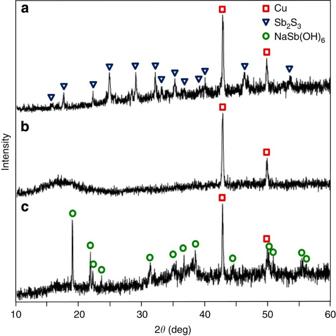Figure 4: Structural changes of rGO/Sb2S3before and after sodiation. X-ray diffractograms of (a) as-coated anode, (b) discharged to 0 V and (c) discharge to 0 V then exposed in air for 48 h. Figure 4 shows the XRD results for the as-coated electrode (a) and the one discharged to 0 V (b). The as-coated electrode shows crystalline Sb 2 S 3 diffraction pattern. When the electrode is discharged, no crystalline phase can be observed, suggesting that the material becomes amorphous. No crystalline phase is observed also for the electrode half discharged to 1 V (case (i)), and the electrode fully discharged to 0 V and then charged to 2 V (case (iii)), suggesting breakdown of the crystal structure after charge and discharge. If the discharged electrode (to 0 V) is exposed to air for 48 h ( Fig. 4c ), crystalline peaks corresponding to NaSb(OH) 6 appears, which is due to the reaction between the discharged material with water and oxygen in the atmosphere. This indicates that Na is incorporated in the electrode after discharging. Figure 4: Structural changes of rGO/Sb 2 S 3 before and after sodiation. X-ray diffractograms of ( a ) as-coated anode, ( b ) discharged to 0 V and ( c ) discharge to 0 V then exposed in air for 48 h. Full size image SEM images of the as-coated and discharged electrodes are shown in Fig. 5 . The as-coated electrode ( Fig. 5a ) shows some small particles on the surface, which is identified as elemental sulphur in energy-dispersive X-ray analysis. During the synthesis process, a small amount of residual sulphur is produced as a by-product, as suggested by previous X-ray photoemission spectroscopy measurements [24] . Upon discharging to 0 V, large elongated particles are observed on the electrode ( Fig. 5b ). Energy-dispersive X-ray analysis shows that the particles have an atomic ratio of Na to S of 2:1, consistent with the formation of Na 2 S from the reaction mechanism. 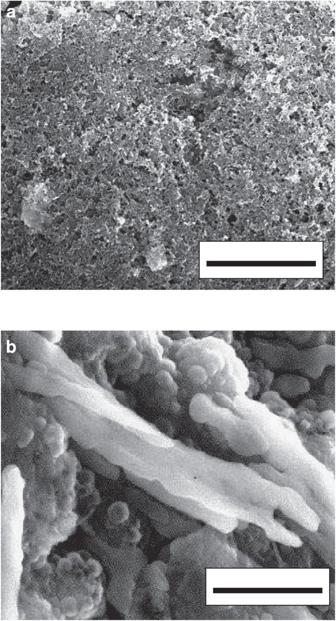Figure 5: Morphological changes of rGO/Sb2S3electrode before and after sodiation. SEM images of the surface of (a) the as-coated electrode and (b) the electrode discharged to 0 V (scale bar, 10 μm). Figure 5: Morphological changes of rGO/Sb 2 S 3 electrode before and after sodiation. SEM images of the surface of ( a ) the as-coated electrode and ( b ) the electrode discharged to 0 V (scale bar, 10 μm). Full size image By anchoring Sb 2 S 3 nanocrystalline on graphene sheet, we were able to design an excellent anode material for NIBs that combines both the high capacity offered by Sb 2 S 3 as well as the stable cycle performance and good rate performance from the graphene template. Capacity and rate capability are the highest so far recorded for anodes in NIBs. To demonstrate the feasibility of rGO/Sb 2 S 3 in a Na metal-free battery, full cell test by coupling rGO/Sb 2 S 3 anode and Na 2/3 Ni 1/3 Mn 2/3 O 2 cathode was carried out. Na 2/3 Ni 1/3 Mn 2/3 O 2 has an average potential of about 3.3 V versus Na/Na + and rGO/Sb 2 S 3 average potential is about 1.1 V versus Na/Na + , a full cell with an average voltage of about 2.2 V is obtained (see Methods section for details of the cathode synthesis). 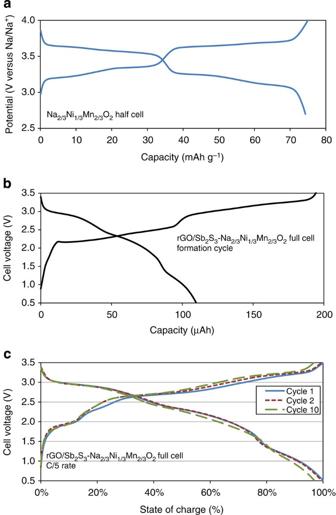Figure 6: Full cell performance of Na metal-free battery with rGO/Sb2S3anode and Na2/3Ni1/3Mn2/3O2cathode. (a) Charge–discharge curves of the Na2/3Ni1/3Mn2/3O2 half cell at 15 mA g−1. (b) Initial charge–discharge of the rGO/Sb2S3and Na2/3Ni1/3Mn2/3O2full cell. (c) Charge and discharge curves for the 1st, 2nd and 10th cycle after the formation cycle. Thexaxis is converted to state of charge (with respect to 110 μAh) to allow easier comparison. Figure 6a shows the charge–discharge profiles of the Na 2/3 Ni 1/3 Mn 2/3 O 2 cathode. A reversible capacity for the cathode of 75mAh g −1 is obtained between 2.7 and 4.0 versus Na/Na + , which is consistent with those results from the literature [26] , [27] . A full cell with a theoretical capacity of 210 μAh was constructed using rGO/Sb 2 S 3 anode and Na 2/3 Ni 1/3 Mn 2/3 O 2 cathode. The full cell was charged and discharged between a voltage of 0.5 and 3.5 V. Figure 6b shows the initial charge–discharge of the full cell. Initial charge capacity is close to 200 μAh after charging to 3.5 V, which is close to the amount of Na in the cathode. The first discharge capacity of the full cell is 110 μAh with an average potential of 2.18 V, and the primary loss is from the irreversible capacity of the anode. The full cell can be cycled with small amount of degradation. Charge–discharge curves remain similar after 10 cycles (see Fig. 6c ). Figure 6: Full cell performance of Na metal-free battery with rGO/Sb 2 S 3 anode and Na 2/3 Ni 1/3 Mn 2/3 O 2 cathode. ( a ) Charge–discharge curves of the Na 2/3 Ni 1/3 Mn 2/3 O2 half cell at 15 mA g −1 . ( b ) Initial charge–discharge of the rGO/Sb 2 S 3 and Na 2/3 Ni 1/3 Mn 2/3 O 2 full cell. ( c ) Charge and discharge curves for the 1st, 2nd and 10th cycle after the formation cycle. The x axis is converted to state of charge (with respect to 110 μAh) to allow easier comparison. Full size image The energy density of the full cell is calculated to be 80 Wh kg −1 (based on the total mass of the cathode and anode active materials; see Methods for calculation details). This value is a lower limit of the rGO/Sb 2 S 3 –Na 2/3 Ni 1/3 Mn 2/3 O 2 system because our test cell was not optimized. With optimization, the first cycle efficiency can be improved and we expect the energy density can be increased to 100 Wh kg −1 . In addition, if other cathode material such as Na 3 V 2 (PO 4 ) 2 F 3 [28] , Na 3 V 2 (PO 4 ) 3 [29] or NaFe 0.5 Co 0.5 O 2 [30] , with capacity >115 mAh g −1 is used, energy density could be further increased to >150 Wh kg −1 by reducing the amount of cathode materials. For comparison, a LiFePO 4 –Li 4 Ti 5 O 12 LIB system has a voltage of 1.9 V, in which cathode and anode contribute about 150 mAh g −1 each. This corresponds to an energy density per total active material of 142 Wh kg −1 . Thus, our NIB has the potential to reach or even exceed some of the current LIB systems. Synthesis and characterization of rGO/Sb 2 S 3 Details of the material synthesis are recently reported [24] and each intermediate was carefully characterized. Briefly, the synthesis is based on the dissolution of antimony hydroxide in aqueous tetramethylammonium hydroxide under moderate heating and addition of this precursor to aqueous GO dispersion in 20% hydrogen peroxide. Precipitation of the resulting peroxoantimonate onto the GO surface was achieved by addition of ethanol–diethyl ether antisolvent mixture. The peroxoantimonate@GO was sulphurized in alcohol suspension, without reduction of the Sb(V) or formation of antimony sulphide, by bubbling hydrogen sulphide. The sulphur-coated antimony (V) oxide@GO was washed and heat-treated in vacuum at 300 °C in a tube furnace for 5 h to reduce the graphene and antimony to form the rGO/Sb 2 S 3 composite. The as-synthesized materials were characterized by powder XRD to confirm the crystalline Sb 2 S 3 formation. The carbon content of the composite determined by elemental analysis is 17 wt%. Electrode fabrication Both commercial bulk Sb 2 S 3 (Sigma-Aldrich) and rGO/Sb 2 S 3 were used as the active materials. Each material was mixed together with acetylene black (Alfa Aesar) and CMC sodium salt (Sigma-Aldrich) in de-ionized water in a weight ratio of 6:2:2 to make a slurry. The slurry was then coated on copper current collector to make an electrode. The electrode was compressed by a roll press, dried at 110 °C for 4 h in vacuum and then made into 2016 coin cells for testing. Typical thickness of the electrodes is 25–30 μm with a packing density of about 1 g cm −3 . One molar NaClO 4 in propylene carbonate with 5 wt% FEC was used as the electrolyte. Reference electrodes with Cu:AB:CMC and graphene:AB:CMC=6:2:2 were also tested for comparison. Full cell investigations In order to investigate the potential of rGO/Sb 2 S 3 in a Na metal-free battery, full cell test by coupling rGO/Sb 2 S 3 anode and Na 2/3 Ni 1/3 Mn 2/3 O 2 cathode was carried out. The Na 2/3 Ni 1/3 Mn 2/3 O 2 cathode material was synthesized by co-precipitation method with nickel and manganese nitrates in stoichiometric amount with ammonium hydroxide. NaOH was added afterwards as the sodium source. The precursors were then annealed initially at 600 °C for 4 h, ground and re-annealed at 900 °C for 10 h. The cathode material was first tested with Na metal counter to evaluate its capacity. To ensure the reversibility of the cathode material, the potential range of the cathode test was limited to 2.7–4.0 versus Na/Na + . The current rate for the test was 15 mA g −1 . For the full cell, because of the difference in specific capacities of the anode and the cathode, the mass of the electrodes have to be matched. A cathode with a 2.8 mg active mass was used for the test. The initial content of Na in the cathode is therefore 2.8 mg × 75 mAh g −1 =210 μAh. The anode active mass was set at 0.2 mg. The full cell was charged and discharged between a voltage of 0.5 and 3.5 V. Energy density is calculated based on the total cathode and anode active material mass of 3.0 mg at 2.18 V voltage, which gives 80 Wh kg −1 . How to cite this article: Yu, D. Y. W. et al. High-capacity antimony sulphide nanoparticle-decorated graphene composite as anode for sodium-ion batteries. Nat. Commun. 4:2922 doi: 10.1038/ncomms3922 (2013).